Structure of p15PAF–PCNA complex and implications for clamp sliding during DNA replication and repair The intrinsically disordered protein p15 PAF regulates DNA replication and repair by binding to the proliferating cell nuclear antigen (PCNA) sliding clamp. We present the structure of the human p15 PAF –PCNA complex. Crystallography and NMR show the central PCNA-interacting protein motif (PIP-box) of p15 PAF tightly bound to the front-face of PCNA. In contrast to other PCNA-interacting proteins, p15 PAF also contacts the inside of, and passes through, the PCNA ring. The disordered p15 PAF termini emerge at opposite faces of the ring, but remain protected from 20S proteasomal degradation. Both free and PCNA-bound p15 PAF binds DNA mainly through its histone-like N-terminal tail, while PCNA does not, and a model of the ternary complex with DNA inside the PCNA ring is consistent with electron micrographs. We propose that p15 PAF acts as a flexible drag that regulates PCNA sliding along the DNA and facilitates the switch from replicative to translesion synthesis polymerase binding. The DNA-sliding clamp proliferating cell nuclear antigen (PCNA) is an essential factor in replication and repair that recruits polymerases and other DNA-modifying enzymes to the replication fork [1] . PCNA forms an 86-kDa homotrimeric ring [2] that encircles the DNA and anchors binding partners, preventing them from falling off the genomic template. The ring has an inner diameter of ~35 Å, much wider than the ~24 Å diameter of a DNA duplex in the B-form [3] . Apart from DNA-editing factors, PCNA also interacts with non-enzymatic proteins that regulate cell cycle control and survival [4] , [5] . Many PCNA-interacting proteins bind through the PIP-box, a consensus sequence with the pattern QXXhXXaa , where h is an aliphatic-hydrophobic residue, a aromatic-hydrophobic and X any residue [6] . In all known co-crystal structures, the PIP-box residues bind to the PCNA front-face forming a short amino-terminal (N-terminal) β-strand that interacts with the PCNA C-terminus, a short 3 10 helix placed in a hydrophobic pocket and a carboxyl-terminal (C-terminal) β-strand of variable length that pairs with the PCNA interdomain connecting loop (IDCL) [7] . The recognition surface on PCNA is small, contacting 11–18 residues of the ligand. The regions flanking these tightly bound residues are usually not visible in electron density maps, suggesting that the chain breaks away from the clamp surface. A common feature of the PIP-box region in these proteins is its disordered nature, providing an adaptable, yet specific contact site whose affinity for PCNA can be tuned by subtle changes in the sequence [8] . The PCNA-associated factor p15 (p15 PAF , hereafter named p15) is a nuclear protein with a PIP-box [9] and is involved in the regulation of DNA replication and cell cycle progression by interacting with PCNA [10] , [11] , [12] . Overexpression of p15 correlates with tumour progression and poor prognosis in a number of human cancers [13] , [14] , [15] , [16] . Evidence for p15–PCNA interaction comes from yeast two-hybrid and co-immunoprecipitation experiments, but no structural detail of the direct interaction is known. We have previously shown that p15 is a monomeric intrinsically disordered protein with conformational preferences in certain regions, including the PIP-box [17] . Here we present an extensive characterization of the interaction between p15 and PCNA based on an integrative structural approach. Three p15 molecules bind to the trimeric PCNA ring with low micromolar affinity. The central region of p15, including the PIP-box, is tightly bound to the front-face and inner surface of PCNA, while the N- and C-termini remain predominantly disordered at its back- and front-face, respectively, with transient interactions at the PCNA outer surface. This arrangement is consistent with the protection from degradation by the 20S proteasome particle, which rapidly degrades free p15. Most importantly, we show that p15 binds DNA, mainly through its histone-like N-terminal tail. While PCNA alone does not interact with DNA, p15 binds to PCNA and DNA simultaneously via independent sites. Molecular modelling and electron microscopy show that a ternary complex with both p15 and DNA inside the PCNA ring can form. We discuss the possible implications of these findings for the regulation of DNA replication and repair, and propose that p15 acts as a flexible drag that regulates PCNA sliding along the DNA, facilitating the switch from replicative to translesion synthesis polymerase binding. p15–PCNA interaction involves an extended PIP-box region Changes in the NMR spectra of p15 and PCNA in the presence of each other ( Fig. 1a,b ) confirm a direct interaction between both proteins. Isothermal titration calorimetry (ITC) measurements could be fitted very well to a model assuming independent p15 binding to equivalent sites in the PCNA trimer, with a dissociation constant of 1.1 μM at 25 °C ( Fig. 1c ). Thus, three p15 molecules bind to the three PCNA protomers, with no indication of cooperativity. The enthalpic contribution to the free energy is large, but so is the entropic cost, in line with a loss in p15 conformational freedom on binding to PCNA. 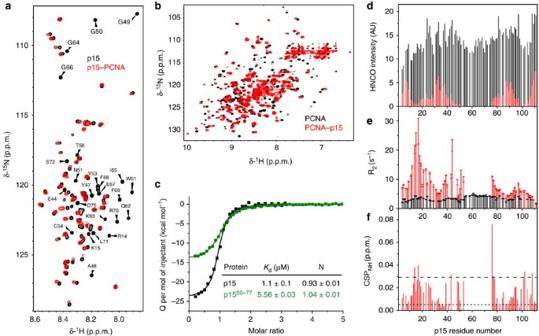Figure 1: The central region of p15 directly binds PCNA with low micromolar affinity. (a) Overlay of1H-15N HSQC spectra of p15 (backbone amide region) in the absence (black) or presence (red) of PCNA at 1:4.2 molar ratio. Signals with strong intensity reduction on binding are labelled. (b) Overlay of1H-15N TROSY spectra of PCNA in the absence (black) or presence (red) of p15 at 1:3.3 molar ratio. (c) ITC curves of p15 (black) and p1550–77(green) binding to PCNA at 25 °C. The disociation constant (Kd) and stoichiometry (N) were derived from the fitting (lines) of the experimental data (squares) to a binding model assuming equivalent sites on PCNA. (d) NMR signal intensities from the 3D HNCO spectrum of p15 in the absence (black) or presence (red) of PCNA. Absolute errors in intensities are less than 0.2% of the largest intensity in each spectrum. (e) Transverse15N R2relaxation rates of p15 in the absence (black) or presence (red) of PCNA measured at 25 °C and 101.4 MHz. (f) CSP of p15 backbone amide signals (weighted average for1HNand15N) caused by the presence of PCNA. Dotted and dashed lines indicate the experimental error and average CSP plus one s.d., respectively. Figure 1: The central region of p15 directly binds PCNA with low micromolar affinity. ( a ) Overlay of 1 H- 15 N HSQC spectra of p15 (backbone amide region) in the absence (black) or presence (red) of PCNA at 1:4.2 molar ratio. Signals with strong intensity reduction on binding are labelled. ( b ) Overlay of 1 H- 15 N TROSY spectra of PCNA in the absence (black) or presence (red) of p15 at 1:3.3 molar ratio. ( c ) ITC curves of p15 (black) and p15 50–77 (green) binding to PCNA at 25 °C. The disociation constant (K d ) and stoichiometry (N) were derived from the fitting (lines) of the experimental data (squares) to a binding model assuming equivalent sites on PCNA. ( d ) NMR signal intensities from the 3D HNCO spectrum of p15 in the absence (black) or presence (red) of PCNA. Absolute errors in intensities are less than 0.2% of the largest intensity in each spectrum. ( e ) Transverse 15 N R 2 relaxation rates of p15 in the absence (black) or presence (red) of PCNA measured at 25 °C and 101.4 MHz. ( f ) CSP of p15 backbone amide signals (weighted average for 1 H N and 15 N) caused by the presence of PCNA. Dotted and dashed lines indicate the experimental error and average CSP plus one s.d., respectively. Full size image As a disordered protein, p15 yields NMR spectra with sharp signals and poor dispersion in the proton frequency. On addition of excess PCNA, signal intensities decrease generally and most notably for the central residues V53-D75 that even disappear ( Fig. 1d ). This observation highlights the central region of p15 as the principal binding site for PCNA, which includes the PIP-box motif ( 62 Q KG I GE FF 69 , conserved residues underlined). The p15 NMR signals still visible in the complex retain their low dispersion, indicating that they remain largely disordered and flexible. Nevertheless, in the presence of PCNA, two segments in the N- and C- terminal regions of p15 around the conserved basic residues R14K15 and P100, respectively, show significantly reduced signal intensities ( Fig. 1d ) and increased 15 N R 2 relaxation rates ( Fig. 1e ). While all R 2 rates increase due to the larger molecular size, their abnormal increase in these two regions indicates some conformational restrictions in the complex. Both regions contain clusters of positively charged amino acids that might interact transiently and unspecifically with the negatively charged PCNA surface. In line with this, chemical shift perturbations (CSP) here are the largest observed outside the core binding site ( Fig. 1f ), but still so small that only weak transient interaction is expected. Changes in the NMR spectrum of PCNA on p15 binding are extensive ( Fig. 1b ), more than seen when bound to a PIP-box fragment of p21 CIP1 (hereafter named p21) [18] , suggesting a larger binding area for p15. To study the role of different p15 regions in the interaction with PCNA, we designed three p15 fragments: the N-terminal deletion mutant p15 32–111 (hereafter named p15 ΔN ) lacking many of the residues experiencing reduced NMR signal intensity and enhanced 15 N R 2 rates on PCNA binding; the p15 50–77 fragment comprising the central residues that experience the largest drop in NMR signal intensity on PCNA binding; and p15 59–70 that corresponds to the smallest PIP-box containing fragment of p21 with reported binding to PCNA [19] . All three p15 fragments bind PCNA, but with decreasing affinity ( Supplementary Fig. 1 and Supplementary Table 1 ). The N-terminal deletion mutant binds PCNA with only slightly lower affinity than p15, implying that any transient interactions of the N-terminal V2-S31 residues stabilize the complex only marginally. The affinity of p15 50–77 , however, is reduced by a factor of 5 and the shortest core fragment p15 59–70 even by a factor of 33. These results indicate that residues G50-T58 and/or L71-E77 strongly contribute to PCNA binding, which is further enhanced by residues A32-G49. The NMR spectra of PCNA in the presence of the different constructs indicate rather similar binding modes for p15, p15 ΔN and p15 50–77 , but less so for p15 59–70 ( Supplementary Fig. 2 ). The strong intensity reduction in many PCNA signals in the presence of p15 (and to a lesser extent in the presence of p15 ΔN ) most likely derives from line broadening caused by the increased size of the complex (125 kDa) and by transient interactions with the p15 chain termini. While we have previously assigned the NMR spectrum of PCNA free and bound to a p21 PIP-box peptide [18] , [20] , p15 excess leads to prohibitively large intensity reduction and line broadening that precluded assignment of the p15-bound PCNA spectrum by triple resonance methods. Instead, we transferred the assignment from free PCNA, based on extrapolation from signal shifting in a titration with p15. In this way, we obtained many plausible quantitative CSP values for PCNA signals on p15 binding and assigned an arbitrary CSP cutoff value where signals of free PCNA had disappeared (due to signal attenuation below the noise level or untraceable shifting; Supplementary Fig. 3 ). CSP projection onto the PCNA structure ( Supplementary Fig. 4 ) reveals that binding of all p15 constructs except the core fragment p15 59–70 affects residues not only within the PIP-box-binding site on the front-face, but also on the inner side of the ring. Structure of the p15–PCNA complex Our attempts to co-crystallize p15 and PCNA were unsuccessful and were most likely hampered by the long flexible p15 termini. In contrast, truncated p15 50–77 co-crystallized with PCNA and diffracted up to 2.65 Å resolution ( Table 1 ). Surprisingly, p15 50–77 was found bound to only two of the three PCNA protomers ( Fig. 2a ), while calorimetry indicated 1:1 stoichiometry and the degenerate NMR spectrum of PCNA showed equivalence of all three protomers both in the absence and presence of p15. This discrepancy arises from the crystal packing, where a symmetry-related PCNA molecule occludes the peptide binding site on one protomer ( Supplementary Fig. 5 ). Residues N51-L71 of p15 50–77 are well defined in the crystal structure ( Supplementary Fig. 6 ), although the side chains of N51, R70 and L71 could not be reliably modelled ( Fig. 2b ). The backbone conformation of the two bound peptides is very similar (C α root mean squared deviation=0.32 Å), while the electron density map is better defined for chain D (as named in the Protein Data Bank deposited coordinate file), which is therefore used for the structure discussion hereafter. Table 1 X-ray diffraction data collection and refinement statistics. 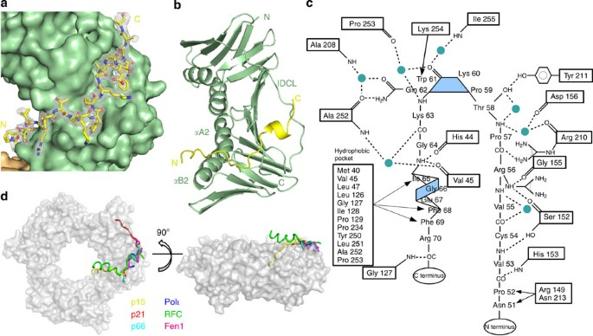Figure 2: Crystal structure of the p1550–77–PCNA complex. (a) Surface representation of one of the three p1550–77-binding sites on the PCNA ring, with the bound p1550–77shown in sticks coloured by atom type. The omit 2F0–FCelectron density map is displayed at 1.2σ. N- and C-termini of p1550–77are indicated. (b) Ribbon diagram of one PCNA protomer (green) with bound p1550–77(yellow). The IDCL and helices αA2 and αB2 (at the inner surface of the PCNA ring) are labelled. (c) Scheme of interactions between p1550–77and PCNA. Indicated are the residue names (framed for PCNA), bound water molecules (blue circles), hydrogen bonds (dotted lines) and non-bonded interactions (arrows). The 310helix and type-I β-turn structures in the bound p1550–77are shaded blue. (d) Front and side views of the PCNA ring (grey surface) with superposed backbones of bound PIP-box fragments from six co-crystal structures: p1551–71(yellow; PDB: 4D2G), p21143–160(red; PDB: 1AXC), Polδ p66453–465(cyan; PDB: 1U76), Polι421–429(blue; PDB: 2ZVM), yeast RFC389–406(green; PDB:1SXJ) and Fen1336–348(magenta; PDB:1U7B). Only the N-terminus of the p15 fragment is found to contact the inner surface of the ring. Full size table Figure 2: Crystal structure of the p15 50–77 –PCNA complex. ( a ) Surface representation of one of the three p15 50–77 -binding sites on the PCNA ring, with the bound p15 50–77 shown in sticks coloured by atom type. The omit 2F 0 –F C electron density map is displayed at 1.2 σ . N- and C-termini of p15 50–77 are indicated. ( b ) Ribbon diagram of one PCNA protomer (green) with bound p15 50–77 (yellow). The IDCL and helices αA2 and αB2 (at the inner surface of the PCNA ring) are labelled. ( c ) Scheme of interactions between p15 50–77 and PCNA. Indicated are the residue names (framed for PCNA), bound water molecules (blue circles), hydrogen bonds (dotted lines) and non-bonded interactions (arrows). The 3 10 helix and type-I β-turn structures in the bound p15 50–77 are shaded blue. ( d ) Front and side views of the PCNA ring (grey surface) with superposed backbones of bound PIP-box fragments from six co-crystal structures: p15 51–71 (yellow; PDB: 4D2G), p21 143–160 (red; PDB: 1AXC), Polδ p66 453–465 (cyan; PDB: 1U76), Polι 421–429 (blue; PDB: 2ZVM), yeast RFC 389–406 (green; PDB:1SXJ) and Fen1 336–348 (magenta; PDB:1U7B). Only the N-terminus of the p15 fragment is found to contact the inner surface of the ring. Full size image The PIP-box residues of p15 50–77 bind to the same groove on the front-face of the PCNA ring as the p21 PIP-box peptide [7] . The side chain of Q62 is hydrogen bonded to PCNA-A252 and, via a water molecule, to PCNA-A208; residues I65-F67 form a short 3 10 helix, and the conserved hydrophobic trident formed by I65, F68 and F69 inserts into the hydrophobic cleft across the N- and C-terminal domains of the PCNA protomer ( Fig. 2c ). Contrary to p21, the residues C-terminal to the p15 50–77 PIP-box do not form a stable intermolecular anti-parallel β-strand with the IDCL of PCNA. Yet the major structural difference to p21 and other PCNA-bound ligands involves residues N-terminal to the p15 50–77 PIP-box and concerns both the peptide conformation and the interaction surface on PCNA. Residues P59-Q62 form a type-I β-turn that reverses the peptide chain direction and sets the N-terminal residues N51-T58 to contact the inner surface of the PCNA ring where they are anchored to a groove between PCNA helices αA2 and αB2 through a network of intermolecular contacts, including five direct and three water-mediated hydrogen bonds ( Fig. 2c and Supplementary Fig. 7 ). Contrarily, in the crystal structures of other PIP-box peptides only a few of the residues N-terminal to the PIP-box are visible, and those seen adopt a different conformation directing the chain away from the PCNA surface ( Fig. 2d ). The orientation of the p15 50–77 peptide chain bound to PCNA in our crystal structure suggests that, in solution, the N-terminal region of full-length p15 passes through the clamp channel to emerge on the back-face of the ring. This conclusion is consistent with the NMR signal perturbations observed for residues at the inner side of the PCNA ring on p15 addition ( Supplementary Fig. 4 ). We furthermore observed several residues on the back-face with perturbed NMR frequencies and/or intensities. Some of them experience small frequency shifting along the titration with p15 (like residue A194 in Supplementary Fig. 8a ), while others do not shift but their intensities decay, vanishing at PCNA:p15 ratios of about 1:0.5 (like residues A82, E143 and K110 shown in Supplementary Fig. 8a ) due to transient p15 contacts at the PCNA back-side. Protein aggregation can be ruled out as an alternative explanation for the signal decay, as confirmed by analytical size exclusion chromatography ( Supplementary Fig. 8b ). Rapid NMR signal decay at substoichiometric ratios without signal reappearance at ligand saturation has also been reported for other protein complexes involving weak transient interactions between charged surfaces [21] or a multitude of binding states [22] . For p15-bound PCNA at the end point of the titration, we observe new signals in the vicinity of some of the vanished ones, but signal broadening and attenuation in the p15–PCNA complex made their unambiguous assignment impossible even with TROSY-based triple resonance experiments [23] . We therefore quantified PCNA signal intensities at substoichiometric PCNA:p15 ratios, where signal positions are still largely as in the free form with selective intensity reduction for signals affected by p15 binding. Since assignment of the NMR signals in this sample is unambiguous, we can confidently project signal attenuations onto the PCNA structure to derive the extended binding surface for full-length p15 ( Fig. 3a ). In agreement with the crystal structure of PCNA bound to the p15 50–77 fragment, the binding site includes residues at the canonical PIP-box-binding groove on the front-face of the ring and extends to helices αA2 and αB2 at its inner surface. Moreover, several PCNA back-face residues also show significant signal attenuation and form a nearly contiguous region. These additional signal attenuations are not observed in the presence of substoichiometric amounts of the truncated p15 50–77 ( Supplementary Fig. 9 ), and indicate a binding mode in which the full-length p15 N terminus passes though the PCNA ring. 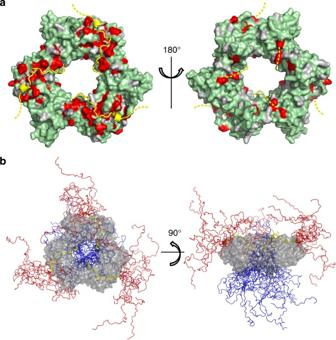Figure 3: Model of the full-length p15–PCNA complex. (a) Surface representation of PCNA (green) with bound p15 (yellow ribbon) showing the front (left) and back (right) face of the ring. The p1550–77–PCNA co-crystal structure with two bound peptide molecules was used as template and complemented by a third p15 peptide (in line with the ITC-derived stoichiometry). The locations of the disordered N- and C-termini are indicated by dashed ribbons. PCNA residues showing NMR signal attenuation in the presence of substoichiometric amounts of p15 (with relative TROSY signal intensity lower than the average minus one s.d.) are coloured red. PCNA residues whose NMR signal intensity could not be reliably measured and prolines are shown in grey. (b) Front and side views of 10 modelled p15–PCNA complex structures consistent with the experimental data. PCNA is shown as grey surface and p15 as ribbons, with the regions seen in the p1550–77–PCNA crystal structure coloured yellow and the added disordered N- and C-terminal extensions in red and blue, respectively. In one of the 10 selected complex models, one p15 N terminus folds back towards the front-face of PCNA instead of passing through the clamp, roughly representing the distribution found in the set of 5,000 modelled complexes. Figure 3: Model of the full-length p15–PCNA complex. ( a ) Surface representation of PCNA (green) with bound p15 (yellow ribbon) showing the front (left) and back (right) face of the ring. The p15 50–77 –PCNA co-crystal structure with two bound peptide molecules was used as template and complemented by a third p15 peptide (in line with the ITC-derived stoichiometry). The locations of the disordered N- and C-termini are indicated by dashed ribbons. PCNA residues showing NMR signal attenuation in the presence of substoichiometric amounts of p15 (with relative TROSY signal intensity lower than the average minus one s.d.) are coloured red. PCNA residues whose NMR signal intensity could not be reliably measured and prolines are shown in grey. ( b ) Front and side views of 10 modelled p15–PCNA complex structures consistent with the experimental data. PCNA is shown as grey surface and p15 as ribbons, with the regions seen in the p15 50–77 –PCNA crystal structure coloured yellow and the added disordered N- and C-terminal extensions in red and blue, respectively. In one of the 10 selected complex models, one p15 N terminus folds back towards the front-face of PCNA instead of passing through the clamp, roughly representing the distribution found in the set of 5,000 modelled complexes. Full size image We then independently generated a large ensemble of p15–PCNA complex structures based only on the p15 50–77 –PCNA crystal structure with randomly appended p15 chain termini. In 98% (92%) of these model complexes, at least one (two) p15 chains pass through the ring. Only 13% of the complexes show all three p15 chains crossing through the ring, presumably due to steric crowding inside the hole that results from building disordered chains randomly. Overall, these results indicate that the conformation of the tightly bound central region of p15 imposes a strong tendency on the p15 N-terminus to pass through the ring. From this ensemble we selected structures where N-terminal p15 residues lie close to the back-face PCNA residues with significantly reduced NMR signal intensity. Ninety-two per cent of complex structures in this subset showed all three p15 chains passing through the PCNA ring and emerging on its back-face, while the remaining modelled complex structures had at least one p15 chain fold back its N-terminus to the PCNA front-face instead of funneling through the ring. A small set of complex model structures illustrating these findings is shown in Fig. 3b . Thus, while the NMR signal attenuations cannot be converted into exact populations of distinct p15 conformations, our results suggest that many (or most) of the p15 N-termini emerge at the back-face of PCNA. The models furthermore suggest that R41-E44 are those p15 residues that most likely contact the PCNA back-face. In line with this, the K42 NMR signal is attenuated beyond detection, A43 shows a significant CSP and E44 a high 15 N R 2 rate in the presence of excess PCNA ( Fig. 1d–f ). Ubiquitin-independent proteasomal degradation of p15 The ubiquitin ligase anaphase-promoting complex/cyclosome and its co-activator Cdh1 target p15 for proteasomal degradation through its conserved KEN-box motif [10] . This mechanism involves recognition of polyubiquitin by the regulatory 19S cap subunits of the 26S proteasome and substrate unfolding by its ATPase subunits before proteolysis within the chamber of the 20S proteasome subcomplex. We found that p15 could also be degraded by the 20S proteasome independent of ubiquitin and ATP, most likely due to its intrinsically disordered state. This degradation is strongly and specifically inhibited in the presence of PCNA ( Fig. 4a ), despite most of the p15 chain remaining flexible and disordered in the bound form. The measured degradation rate is lower than calculated assuming that p15 can only be degraded when dissociated from PCNA ( Fig. 4b ). This reduction indicates that p15 is less accessible to the proteasome even when dissociating from PCNA, possibly because part of it remains trapped within the PCNA ring. 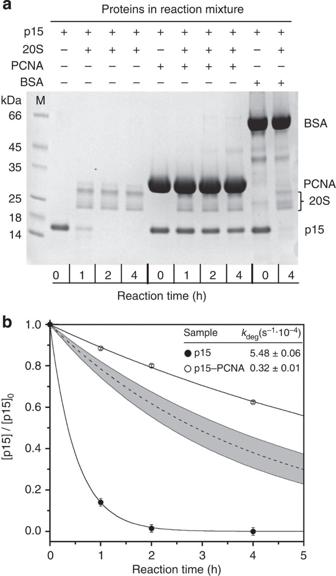Figure 4: Ubiquitin- and ATP-independent degradation of p15 by the 20S proteasome. (a) SDS–PAGE of different reaction mixtures and times, as indicated. The left lane contains the molecular weight markers. (b) Densitometric analysis of SDS–PAGE stains showing the p15 degradation by the 20S proteasome. Filled and open circles show the fraction of p15 remaining after the indicated incubation times with 20S proteasome in the absence and presence of fivefold molar excess of PCNA, respectively. The data were averaged over two independent experiments and fitted to a monoexponential decay (solid lines). The dashed line represents the fraction of remaining p15 calculated assuming that its dissociation from PCNA is not rate limiting for degradation, with the maximal variation (from estimated experimental uncertainty, see Methods) indicated in grey. The values of the degradation ratekdegconsidering this maximal variation are between 0.55 and 0.82·10−4s−1. Figure 4: Ubiquitin- and ATP-independent degradation of p15 by the 20S proteasome. ( a ) SDS–PAGE of different reaction mixtures and times, as indicated. The left lane contains the molecular weight markers. ( b ) Densitometric analysis of SDS–PAGE stains showing the p15 degradation by the 20S proteasome. Filled and open circles show the fraction of p15 remaining after the indicated incubation times with 20S proteasome in the absence and presence of fivefold molar excess of PCNA, respectively. The data were averaged over two independent experiments and fitted to a monoexponential decay (solid lines). The dashed line represents the fraction of remaining p15 calculated assuming that its dissociation from PCNA is not rate limiting for degradation, with the maximal variation (from estimated experimental uncertainty, see Methods) indicated in grey. The values of the degradation rate k deg considering this maximal variation are between 0.55 and 0.82·10 −4 s −1 . Full size image DNA-binding activity of p15 PCNA is loaded on DNA by the clamp loader, which binds, opens, and closes the ring under ATP hydrolysis [24] . Although the inner surface of the ring is lined with helices containing basic residues that complement the negative charge of the DNA backbone, a tight PCNA–DNA interaction is not expected as it would hinder sliding along the DNA. Bacterial [25] and archaeal [26] clamps bind short DNA molecules, but co-crystals of yeast PCNA and a short primed DNA duplex that binds to the bacterial clamp with nM affinity show only weak features within the hole of the ring, interpreted as DNA being highly disordered or having low occupancy [27] . We have analysed the interaction of human PCNA with the same primed DNA in solution by NMR. Even at a high DNA:PCNA molar ratio of 50:1, only very small changes in the 1 H- 15 N NMR signals of PCNA were observed, and affected residues do not localize to any specific area, but are sparsely distributed on the protein surface ( Supplementary Fig. 10 ). This suggests that a direct DNA–PCNA interaction is either absent or extremely weak and unspecific. Several clusters of basic residues in the N- and C-terminal regions of p15 suggest that it may bind DNA through electrostatic interactions. Our modelled structure of the p15–PCNA complex likewise suggests that p15, when brought close to the DNA by binding to a loaded PCNA ring, may bind the DNA with its flexible tails. To test the hypothesis of a p15–DNA interaction, we employed a fluorescence polarization assay and tested DNA sequences reported to bind to S. solfataricus PCNA [26] ( Supplementary Table 2 ). In contrast to its archaeal homologue, human PCNA does not interact with these DNA sequences, while p15 does ( Fig. 5 ). The p15–DNA interaction is unspecific since any of the DNA molecules tested (single-stranded DNA, primed DNA and flapped DNA) are bound by p15 with similar affinity ( Supplementary Fig. 11a ). The binding isotherms could be fitted to a 1:1 interaction model, with apparent dissociation constants between 0.2 and 0.4 μM at 25 °C. Increasing the salt concentration from 40 to 150 mM lowers the affinity by an order of magnitude, indicating that the interaction is predominantly electrostatic ( Supplementary Fig. 11b ). The affinity of p15 ΔN is reduced by two orders of magnitude, indicating that the basic N-terminal region of p15 contributes most to the DNA affinity ( Fig. 5a ). The central fragment p15 50–77 binds DNA with even lower affinity, and no DNA binding was observed with the core PIP-box fragment p15 59–70 . When DNA was titrated with PCNA-bound p15, the increase in fluorescence polarization was larger ( Fig. 5a ), indicating that a ternary complex forms (since the larger the size of the complex the larger the polarization). The slightly reduced DNA affinity shows that PCNA interferes only weakly with p15 binding to DNA. Similarly, when DNA-bound p15 was titrated with PCNA ( Fig. 5b ) the PCNA affinity was comparable to that of isolated p15 (or p15 50–77 ). Thus, a ternary p15–PCNA–DNA complex forms in solution in which the direct p15–PCNA and p15–DNA interactions are largely independent of each other. 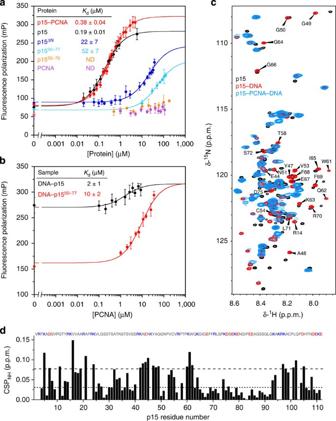Figure 5: DNA-binding activity of p15. (a) Fluorescence polarization of 50 nM fluorescein-labelled flapped DNA in the presence of increasing concentrations of different p15 constructs, PCNA, or a 1:3 (molar ratio) mixture of p15 and PCNA. Measurements (filled circles) were averaged over three independent experiments, with the s.d. indicated by the error bars, and fitted to a binding model assuming 1:1 stoichiometry (lines). (b) Fluorescence polarization of flapped DNA in the presence of 6 μM p15 (black) or 124 μM p1550–77(red), and increasing PCNA concentration. Data analysis was done as ina. (c) Overlay of1H-15N HSQC spectra (backbone amide region) of p15 alone (black), in the presence of dsDNA (red) and in the presence of both dsDNA and PCNA (blue). The three samples contained low salt buffer. (d) CSP of p15 backbone amide signals caused by dsDNA binding in low salt buffer. Dotted and dashed lines indicate the experimental error and average CSP plus one s.d., respectively. The amino acid sequence of p15 is indicated above the plot. Residues with positive charge are coloured blue, negative red and neutral grey. All data were measured at 25 °C. Figure 5: DNA-binding activity of p15. ( a ) Fluorescence polarization of 50 nM fluorescein-labelled flapped DNA in the presence of increasing concentrations of different p15 constructs, PCNA, or a 1:3 (molar ratio) mixture of p15 and PCNA. Measurements (filled circles) were averaged over three independent experiments, with the s.d. indicated by the error bars, and fitted to a binding model assuming 1:1 stoichiometry (lines). ( b ) Fluorescence polarization of flapped DNA in the presence of 6 μM p15 (black) or 124 μM p15 50–77 (red), and increasing PCNA concentration. Data analysis was done as in a . ( c ) Overlay of 1 H- 15 N HSQC spectra (backbone amide region) of p15 alone (black), in the presence of dsDNA (red) and in the presence of both dsDNA and PCNA (blue). The three samples contained low salt buffer. ( d ) CSP of p15 backbone amide signals caused by dsDNA binding in low salt buffer. Dotted and dashed lines indicate the experimental error and average CSP plus one s.d., respectively. The amino acid sequence of p15 is indicated above the plot. Residues with positive charge are coloured blue, negative red and neutral grey. All data were measured at 25 °C. Full size image The interaction of p15 with DNA was further characterized by NMR using a 24 bp duplex ( Supplementary Table 2 ). Perturbations in several p15 resonances confirmed the binding ( Fig. 5c ). The largest CSP occur near clusters of basic residues mainly in the N-terminal half ( Fig. 5d ). Conversely, the smallest perturbations occur near clusters of acidic residues in the C-terminal region. Titration with DNA provokes linear shifts for several p15 NMR signals in medium-salt buffer, but non-linear curved shifts in low-salt buffer ( Supplementary Fig. 12 ). The latter indicates more than one binding site, while linear shifting is consistent with a single binding site [28] . These results confirm the electrostatic nature of the p15–DNA interaction with an affinity in the low micromolar range at physiological ionic strength. The poor H N signal dispersion and only minor changes in C α chemical shifts ( Supplementary Fig. 13 ) indicate that p15 does not acquire a defined structure on binding to the DNA; rather, its backbone remains flexible and disordered. In the presence of PCNA, DNA-bound p15 shows a similar pattern of NMR signal attenuation as in the absence of DNA ( Fig. 5c ), in line with a ternary complex where the central region of p15 is tightly bound to PCNA. To assess whether a DNA duplex could fit inside the p15-bound PCNA ring, we built models based on the crystal structure of the p15 50–77 –PCNA complex with the p15 N- and C-termini protruding from opposite faces of the PCNA ring. 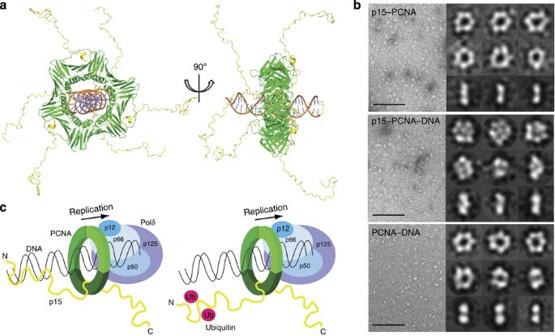Figure 6: Model of the ternary p15–PCNA–DNA complex. (a) Ribbon plot of PCNA (green), p15 (yellow) and a regular B-form 24 bp DNA duplex (orange and blue). (b) Electron microscopy pictures of the mixtures with negative staining. Representative areas of digital micrographs are shown at the left, selected class averages resulting from 2D reference-free alignment at the right (top-, tilted- and side-views from top to bottom). The bars drawn on each of the three micrographs are 100 nm long. (c) Scheme for a possible arrangement of the PCNA ring sliding along the DNA, with the replication polymerase δ complex bound at the front-face. In this model, one p15 chain traverses the clamp channel, with its N-terminal tail binding the DNA at the back-face of PCNA. This p15–DNA interaction could be disrupted by p15 ubiquitylation at K15 and K24 occurring during S-phase progression and, thus, modulate PCNA diffusion along the DNA. Figure 6a shows that formation of such a complex is possible from steric and energetic considerations ( Supplementary Fig. 14 ). For an experimental verification of this possibility, PCNA in the presence of p15, DNA or both was stained with uranyl acetate and observed by transmission electron microscopy ( Fig. 6b ). Two-dimensional analysis of single particle projections yielded class averages for top-, side-, and tilted-views of the PCNA ring, with a larger proportion of tilted-view classes for the ternary p15–DNA–PCNA complex ( Supplementary Fig. 15 ). Most remarkably, many of the top- and tilted-views of the ternary complex show increased density within the PCNA ring compared to both binary mixtures (where only the p15–PCNA mixture, however, is expected to form a complex). The same result is obtained when the rotational power spectra of individual particles in the three data sets are calculated and classified ( Supplementary Fig. 16 ). These observations indicate that p15-bound DNA in the ternary complex is (at least transiently) located within the PCNA ring. The micrographs do not inform about the location of p15, and we cannot confirm whether p15 passes through the centre of PCNA also in the ternary complex. However, the high similarity in the pattern of p15 NMR signals that vanish when bound to PCNA both in the presence and in the absence of DNA ( Figs 1a and 5c ) indicates that the structure of the tightly bound region is the same, with its N-terminus oriented towards the back-face, suggesting that it passes through the ring as in the binary p15–PCNA complex. Figure 6: Model of the ternary p15–PCNA–DNA complex. ( a ) Ribbon plot of PCNA (green), p15 (yellow) and a regular B-form 24 bp DNA duplex (orange and blue). ( b ) Electron microscopy pictures of the mixtures with negative staining. Representative areas of digital micrographs are shown at the left, selected class averages resulting from 2D reference-free alignment at the right (top-, tilted- and side-views from top to bottom). The bars drawn on each of the three micrographs are 100 nm long. ( c ) Scheme for a possible arrangement of the PCNA ring sliding along the DNA, with the replication polymerase δ complex bound at the front-face. In this model, one p15 chain traverses the clamp channel, with its N-terminal tail binding the DNA at the back-face of PCNA. This p15–DNA interaction could be disrupted by p15 ubiquitylation at K15 and K24 occurring during S-phase progression and, thus, modulate PCNA diffusion along the DNA. Full size image We have used an integrative structural approach to characterize the interaction of the intrinsically disordered protein p15 with the DNA-sliding clamp PCNA. By NMR, we identified the p15 core interaction region and designed a p15 50–77 fragment with truncation of the flexible tails that impeded crystallization of the full-length p15–PCNA complex. The well-diffracting p15 50–77 –PCNA crystals reveal interactions also outside the canonical PIP-box that reach into the PCNA ring and substantially contribute to the binding free energy. ITC measurements also confirm that one p15 molecule binds to each of the three protomers in the PCNA ring with low μM affinity, although our crystal structure shows only two bound p15 50–77 molecules due to a crystal packing artifact. The non-cooperative 1:1 stoichiometry is common to all PIP-box containing proteins whose binding to PCNA has been studied by calorimetry [19] , [29] . The mode of p15 binding to PCNA, however, differs importantly in that p15 extends its interaction site N-terminally from the PIP-box-binding groove on the front-face to the inner surface of the PCNA ring. Both the backbone orientation of the p15 50–77 N terminus visible in the crystal structure and the NMR data with full-length p15 strongly suggest that the flexible N-terminus passes through the PCNA ring to emerge, and transiently contact, on its back-face. In the ensemble of p15–PCNA complexes modelled from these findings, most of the bound p15 chains have their flexible N- and C-termini protrude at the opposite back and front faces of the PCNA ring, respectively ( Fig. 3b ). In the nucleus of the cell, the various PCNA ligands compete for binding to the three protomers of the ring and there likely is a hierarchy based on relative affinities modulated by post-translational modifications that, together with steric hindrance and relative protein concentrations, determine the occupancy of the PCNA protomers [30] . The simultaneous occupation of all three sites by identical ligands, as seen here and in other quantitative binding studies, may not be the prevalent situation inside the cell. Only the small and disordered p21 protein might have an affinity high enough to displace any other ligand from PCNA, explaining its dominant inhibition of DNA replication and cell cycle progression [31] . For instance, a C-terminal p21 fragment [32] binds PCNA with two orders of magnitude higher affinity than p15. Conversely, the affinity of PCNA for p15 is higher than for a PIP-box fragment of the p66 subunit of the replicative polymerase δ (Polδ; K d =15.4 μM, measured by ITC at 30 °C) [29] , and similar to the translesion synthesis polymerase η (TLS Polη; K d =0.4 μM, measured by surface plasmon resonance at 25 °C) [33] . Polδ is a four-subunit complex of 239 kDa, much larger than PCNA, which possibly occludes (by binding and steric hindrance) more than one PIP-box-binding groove, as observed in the complexes of large proteins with PCNA rings [34] , [35] . Polη is a 78-kDa multidomain protein with an ubiquitin-binding domain that increases its affinity for PCNA when ubiquitylated at K164 after ultraviolet irradiation [36] . The rapid degradation of p15 by the 20S proteasome core particle suggests that this may be a mechanism for regulating free p15 levels in the cell, in addition to the ubiquitin- and ATP-dependent one. PCNA binding, however, strongly inhibits p15 degradation by the 20S proteasome, and the degradation rate is lower than expected if dissociation from PCNA was not rate limiting. Apparently, p15 is less accessible to the proteasome even after dissociation from PCNA, consistent with the modelled complex structure where p15 may stay partly trapped within the PCNA ring. Degradation by the 20S proteasome and its inhibition on binding to PCNA have also been described for p21 (ref. 37 ). A short sequence C-terminal to the p21 PIP-box is essential for binding to one of the α-subunits of the 20S proteasome. Part of this sequence ( 156 RLIFSK 161 ) is tightly bound to PCNA in the crystal structure of the complex and PCNA binding might mask the recognition site. The corresponding sequence, however, is very different in p15 ( 74 KDSEKE 79 ) and is not tightly bound to PCNA. Both p15 and PCNA are primarily expressed during the S-phase of the cell cycle, when chromosomal replication occurs, and both are mainly associated with the chromatin [10] , [11] . Thus, while p15 may be bound to PCNA alone, its functionally relevant form in DNA replication and repair is that bound to the DNA-loaded PCNA. We have found that p15 by itself binds to DNA, predominantly via electrostatic interactions with its basic N-terminal tail. This region contains an 21 APRK [24] sequence similar to the known DNA-binding motif SP(R/K)(R/K) [38] that is present in p15 homologues as well as in the N-terminal histone H3 tail ( Supplementary Fig. 17 ). The flexible N-terminal histone tails are likewise rich in basic residues and have been proposed to unspecifically bind DNA, thus attenuating electrostatic repulsion in the chromatin [39] . While human PCNA alone does not interact noticeably with DNA, p15 can bind to PCNA and DNA simultaneously via independent sites and with similar affinities. Our structure-based model of the ternary complex shows that the PCNA trimer may accommodate up to three p15 molecules plus the duplex DNA within its central cavity ( Fig. 6a ). This model is consistent with our electron micrographs that show the PCNA ring at least partially filled by p15-bound DNA ( Fig. 6b ). On the basis of these observations, we propose that the flexible N-terminal tail of p15 may act as an extended arm that captures and binds the DNA fibre at the back-face of PCNA. It could, thus, modulate and slow down the linear diffusion of PCNA along the DNA ( Fig. 6c ). Since the mean diffusion coefficient of human PCNA sliding along dsDNA is D =1.16 μm 2 s −1 , unrestrained PCNA would diffuse by several hundred bp in a few ms [40] . The E. coli β-clamp binds DNA with nanomolar affinity and has a coefficient of diffusion on DNA that is two orders of magnitude lower than for human PCNA [41] . The processivity subunit of the herpes simplex virus DNA polymerase UL42 likewise has nanomolar affinity for DNA, which is remarkably high for a sequence-independent DNA-binding protein [42] , while the interaction of S. cerevisiae PCNA with DNA is very weak [27] . This comparison suggests a loss in DNA affinity during the evolution of DNA-sliding clamps, with a concomitant gain in processivity that implies faster diffusion along the DNA. In higher organisms, p15 might help to regulate the sliding velocity of PCNA, and this p15 function may be required for the DNA damage response to prevent rapid drift of PCNA at stalled replication forks between DNA polymerase swapping events. Interestingly, a fraction of PCNA-bound p15 is ubiquitylated at K15 and K24 during normal S-phase progression and is selectively degraded by the proteasome after ultraviolet irradiation [11] . The affinity of p15 for DNA would likely be reduced by ubiquitylation of these lysines in the p15 N-terminal region that primarily interacts with the DNA, as it removes positive charges and introduces steric hindrance. Thus, ultraviolet irradiation would shift the equilibrium from ubiquitylated to non-ubiquitylated PCNA-bound p15 that is more competent for DNA binding, and the switch from the replicative polymerases (like Polδ) to TLS polymerases (like Polη) could be facilitated. Our proposed model for p15-modulated PCNA sliding along the DNA could in future be validated by single-molecule experiments [40] . The PIP-box/PCNA interaction is a promising target for cancer therapeutics [43] , [44] . Yet, PCNA directs fundamental DNA-templated processes, and targeting its common interaction site for so many different PIP-box proteins might cause unspecific cytotoxicity. Our studies reveal that p15 exhibits a so-far unique binding mode among PIP-box proteins in which residues N-terminal to the PIP-box contribute importantly by binding on the inside of the PCNA ring. Targeting this novel interaction might provide an avenue to inhibitors with high selectivity for the oncogenic p15. Clones and proteins Human PCNA (UniProt: P12004) was produced in E. coli BL21(DE3) cells grown in appropriate culture media to obtain protein with natural isotopic abundance or uniform enrichment using a clone with N-terminal His 6 -tag and PreScission protease cleavage site in a pET-derived plasmid. For NMR samples, the protein was purified from the soluble fraction by Co 2+ -affinity chromatography, cleaved by PreScission protease, and polished by gel filtration chromatography [45] . The NMR sample buffer was PBS (137 mM NaCl, 2.7 mM KCl, 10 mM sodium phosphate, 2 mM potassium phosphate) pH 7.0. All columns and chromatography systems were from GE Healthcare. Protein elution was monitored by absorbance at 280 nm and confirmed by SDS–polyacrylamide gel electrophoresis (SDS–PAGE). The purified protein contained the extra sequence GSH at the N-terminus. The PCNA sample for crystallization was obtained by introducing two additional purification steps. The sample cleaved with PreScission protease was dialysed against 50 mM sodium acetate pH 5.5, 100 mM NaCl. After separation of some precipitated material, the solution was loaded on a HiTrap Heparin HP column equilibrated with the same buffer. After column washing, the protein was eluted with a 0–100% gradient of 50 mM sodium acetate pH 5.5, 2 M NaCl in 20 column volumes (CV). The protein-containing fractions of the major peak were dialysed against 20 mM Tris-HCl buffer pH 7.6, 150 mM NaCl and injected into a HiTrap Chelating HP column loaded with Co 2+ cations to remove uncleaved PCNA. The flow-through was loaded on a HiTrap Q Sepharose column and eluted with a 0–60% gradient of 20 mM Tris-HCl pH 7.6, 1 M NaCl in 5 CV. The protein-containing fractions were concentrated and polished using a Superdex 200 26/60 column equilibrated with PBS, pH 7.0, and then exchanged into the crystallization buffer (20 mM Tris-HCl, pH 7.5, 10% glycerol, 2 mM dithiothreitol (DTT)) using a PD10 column. Stock solutions in PBS or crystallization buffer were flash-frozen in liquid nitrogen and stored at −80 °C. The protein concentrations were measured by absorbance at 280 nm using the extinction coefficient calculated from the amino acid composition (15,930 M −1 cm −1 ). All indicated concentrations of PCNA samples refer to protomer concentrations. Human p15 (Uniprot: Q15004) was produced using E. coli BL21(DE3) cells grown in the appropriate culture media and purified by three sequential chromatographic separations: anion exchange, reverse phase, and cation exchange [17] . This purified protein does not contain any extraneous residue, but mass spectrometry showed that it lacks the initial methionine. The gene encoding the p15 mutant with residues 2–31 deleted (p15 ΔN ) was generated using the QuikChange Site-Directed Mutagenesis Kit (Agilent). The p15 ΔN –pET11d construct was introduced in E. coli BL21(DE3) cells and grown at 37 °C until OD 600 =0.6, when protein expression was induced with 1 mM isopropyl-β- D -thiogalactoside for 3 h at 37 °C. Cells were harvested and resuspended in lysis buffer (20 mM Tris, pH 8.0, 1 mM DTT, 1 mM EDTA plus one tablet of the protein inhibitor cocktail Complete from Roche) and sonicated on ice. Cells were pelleted by centrifugation at 4 °C at 25,000 r.p.m. for 1 h. After centrifugation, the supernatant was loaded on a Hiload 26/10 Q Sepharose HP column. The column was washed with 20 mM Tris, pH 8.0, 1 mM DTT, 1 mM EDTA (Buffer A) and the protein was eluted with a two-step gradient using buffer A with 2 M NaCl (0–20% in 0.3 CV and 20–100% in 1 CV). Fractions containing the protein, as seen in SDS–PAGE, were pooled, diluted three times in buffer A, and loaded on a HiLoad 26/10 SP Sepharose HP column. The protein was eluted with a 0–51% gradient of buffer B and the fractions containing the protein were concentrated and polished by gel filtration on a Superdex 75 26/60 column previously equilibrated with PBS, pH 7.0, 1 mM DTT. Mass spectrometry analysis of the purified material confirmed the identity of the polypeptide, which lacked the initial methionine of the construct and contained residues 32–111 of human p15. Peptides p15 50–77 ( 50 GNPVCVRPTPKWQKGIGEFFRLSPKDSE 77 ) and p15 59–70 were purchased from Apeptide Co. For NMR, ITC and fluorescence polarization measurements, concentrated peptide stock solutions were prepared dissolving the lyophilized powder in water or in PBS, pH 7.0, and the pH was adjusted with NaOH, if necessary. For crystallization, the buffer was 20 mM Tris, pH 7.5, 0.5 mM TCEP. The peptide concentration was measured by absorbance at 280 nm using the extinction coefficient calculated from the amino acid composition. NMR spectroscopy Unless indicated otherwise, all NMR data were measured on a Bruker Avance III 800 MHz (18.8 T) spectrometer equipped with a cryogenically cooled triple resonance z-gradient probe. 1 H- 15 N TROSY spectra of PCNA were recorded at 35 °C on samples of 50 μM U-[ 2 H, 15 N] PCNA with or without p15 molecules at different concentrations in PBS pH 7.0, 1 mM DTT. The spectra used for assignment of p15 bound to PCNA were recorded at 25 °C on a sample containing 0.15 mM U-[ 13 C, 15 N] p15, 0.75 mM U-[ 2 H] PCNA in PBS, pH 6.9, 1 mM DTT, 5% D 2 O. Assignment of H N , N, C′, C α and C β resonances was obtained from three-dimensional (3D) HNCO, HN(CA)CO, HNCA, HN(CO)CA, HNCACB and HN(CO)CACB spectra, assisted by the previously published free p15 assignment [17] . 1 H chemical shifts were referenced to internal 2,2-dimethyl-2-silapentane-5-sulfonate (DSS, 0.00 p.p.m. ), and 13 C and 15 N chemical shifts were indirectly referenced to DSS [46] . The p15 backbone 15 N R 2 relaxation rates at 25 °C and 101.4 MHz were measured on a Bruker Avance 1 GHz (23.4 T) spectrometer equipped with a cryogenically cooled triple resonance z-gradient probe. A series of two-dimensional 1 H- 15 N correlation maps modulated by different values of the 15 N transverse relaxation delay were acquired in a fully interleaved mode [17] . The samples contained 180 μM U-[ 15 N] p15 in 200 mM MES buffer, pH 6.8, 0.5 mM DTT, 5% D 2 O with or without 750 μM unlabelled PCNA. These two samples were prepared from stocks of p15 and PCNA simultaneously dialysed in the same beaker and buffer, eliminating the possibility for bias in the measured CSP (shown in Fig. 1f ) by differences in pH or ionic strength. CSP values and their errors were computed as the weighted average distance between backbone amide 1 H and 15 N chemical shifts in the free and bound states [47] . NMR titration of PCNA with p15 was performed using stocks of 50 μM 2 H, 15 N-PCNA and 1 mM p15 in PBS, NaN 3 0.02%, pH 7.3 recording 1 H- 15 N TROSY spectra at 35 °C and different PCNA:p15 ratios. Quantitative signal intensity analysis at 1:0.2 ratio was done on 200 μM PCNA samples with 40 μM p15 or p15 50–77 . NMR signals of p15 samples at concentrations between 20 μM and 1 mM did not show any sign of aggregation. Analytical size exclusion chromatography of 50 μM PCNA, 250 μM p15, or the mixture of both, performed at room temperature on a Superdex 200 10/300 GL column, showed, homogenous samples with no indication of aggregation. PCNA binding to the short primed DNA was investigated at 35 °C by comparison of 1 H- 15 N TROSY spectra recorded on a 50-μM U-[ 15 N, 2 H] PCNA in PBS, pH 7.0, with or without 2.5 mM DNA. NMR titrations of p15 with dsDNA in PBS or MES buffer were performed by adding small volumes of highly concentrated DNA stock solutions to p15 samples, such that changes in p15 concentration remained small. Assignment of backbone H N , H α and N chemical shifts of p15 bound to dsDNA in low-salt buffer (20 mM MES, 1 mM DTT, pH 6.1) at 25 °C was obtained from 3D 1 H- 15 N HSQC-TOCSY, 1 H- 15 N HSQC-NOESY and HNHA experiments recorded on a sample containing 30 μM U-[ 15 N] p15 and 42 μM dsDNA. Assignment of the H N , N, C′, C α and C β resonances of p15 bound to dsDNA in medium-salt buffer (PBS, pH 6.3, 1 mM DTT) at 25 °C was obtained from 3D HNCO, HN(CO)CA, HNCA and HN(CO)CACB experiments recorded on a sample containing 50 μM U-[ 13 C, 15 N] p15 and 125 μM dsDNA. Isothermal titration calorimetry These measurements employed an ITC200 calorimeter. Protein solutions (dialysed against PBS, pH 7.0, 2 mM TCEP) were titrated with concentrated peptide stocks prepared by dissolving the lyophilized peptides in the dialysis buffer and adjusting the pH to 7.0 with NaOH, if necessary. The binding isotherms were analysed by non-linear least-squares fitting of the experimental data to a model assuming a single set of equivalent sites [48] . Data analysis employed Microcal Origin (OriginLab) and in-house developed software. Protein crystallization and structure determination Stocks of PCNA and p15 50–77 solutions were mixed to final concentrations of 0.5 mM and 0.6 mM, respectively (1:1.2 monomer molar ratio) and incubated at room temperature for 30 min before screening crystallization conditions by the hanging drop vapour diffusion method. Best diffracting co-crystals grew within 3 days at 18 °C in 2 μl droplets obtained by mixing 1 μl of the complex solution and 1 μl of a solution containing 40% polyethylene glycol 300 in 0.1 M sodium phosphate-citrate buffer pH 4.2. Microseeding with seed beads (Hampton Research) was used to improve the crystals, which were flash-frozen directly from the drops. All data were collected at 100 K using synchrotron radiation ( λ =1.00 Å) at the PXI-XS06A beamline (SLS, Villigen, Switzerland) and a Pilatus 6M detector. Diffraction data processing and scaling was accomplished with X-ray Detector Software (XDS) [49] . The structure of the p15 50–77 –PCNA complex was determined by molecular replacement using Phaser [50] and the previously reported human PCNA structure as a search model (PDB:1VYM). The initial model was positioned manually with Coot [51] and refined using PHENIX [52] . Refinement and data collection statistics are summarized in Table 1 . Protein–DNA hydrogen bonds and Van der Waals contacts were identified and analyzed with the Protein, Interfaces, Surfaces and Assemblies service (PDBePISA) at the European Bioinformatics Institute [53] . Fluorescence spectroscopy Deoxyoligonucleotides for fluorescence polarization experiments were purchased from Thermo Fischer Scientific, and their concentration was determined from the extinction coefficient at 260 nm. The DNA molecules were obtained by mixing equimolar amounts of the appropriate oligonucleotides (indicated in Supplementary Table 2 ) in 20 mM Tris-HCl, pH 7.8, 25 mM NaCl, at 93 °C for 2 min with subsequent slow cooling at room temperature. Binding experiments used samples with 50 nM fluorescein-labelled DNA in 30 mM HEPES, pH 7.6, 40 mM KCl, 5% glycerol, 0.1 g l −1 bovine serum albumin, 2 mM TCEP with increasing concentrations of the different p15 molecules or PCNA. Fluorescence polarization measurements were performed at 25 °C on a FluoroMax-3 spectrometer (Horiba Scientific) with a 10 mm Hellma quartz cuvette using the constant wavelength module for quantitative analysis. The excitation wavelength was 490 nm and the emission wavelength 515 nm. s.d. were calculated from the polarization values of three repeated measurements. Kaleidagraph (Synergy Software) was used to fit the experimental data to a one-site-binding model. Molecular modelling The structure of full-length p15 bound to PCNA was modelled starting from the crystal structure of the p15 50–77 –PCNA complex. The conformation of residues 51 to 71 was maintained as in the crystal structure, and disordered N- and C-terminal extensions were built into each p15 50–77 peptide using Flexible-Meccano [54] to sequentially generate peptide chains based on amino acid specific conformational propensity and volume exclusion with statistical conformation sampling. An ensemble of 100,000 full-length p15 conformers was generated for each of the three bound peptides, and side chains were added to each conformer using SCCOMP [55] . These p15 conformers were then docked individually onto the PIP-box binding site of PCNA and discarded if steric clashes with PCNA were detected, resulting in 11,000 p15 conformers for each of the three equivalent binding sites on the PCNA trimer. These conformers were then randomly selected and docked on the PCNA ring to generate 5,000 models of the complex with three bound p15 chains and no steric clashes between them. Another set of 5,000 models of the complex with three bound p15 chains was generated in the same way but using subsets of the p15 conformers with at least one residue in their N-terminal tails (V2-G50) closer than 6.5 Å (C β −C β distance) to any of those PCNA back-face residues showing reduced TROSY signal intensity in the presence of substoichiometric amounts of p15 (that is, PCNA residues V7, A82, E85, F103, K110 and E143). To classify the p15 chains as crossing the ring or not, the centre of mass of PCNA and a plane passing through this centre and perpendicular to the three-fold symmetry axis of PCNA were defined. A p15 chain was considered to go through PCNA if at least one of the heavy atoms in residues 2–50 fulfils both of the following two criteria: (i) the vector connecting the centre of mass of PCNA and the heavy atom has a positive dot product with the normal to the plane directed to the back-face: (ii) the distance between the heavy atom and the PCNA centre of mass is less than 17 Å (half the diameter of the PCNA ring; to exclude chains that comply with the first criterion but going over the ring instead of through it). To model the ternary p15–PCNA–DNA complex, disordered tails of p15 were added to the p15 50–77 –PCNA crystal structure using Coot [51] , where backbone dihedral angles were adjusted manually to maximize the empty space within the PCNA central cavity. The 24 bp DNA duplex in regular B conformation was then placed within the channel, and the whole ternary complex structure was refined by simulated annealing and energy minimization using loose and ambiguous distance restraints between DNA and PCNA in the HADDOCK refinement protocol [56] . Atoms at the interface (within 6.5 Å) were allowed to sample additional conformations during a semi-flexible simulated annealing, and further refinement in explicit water solvent was performed. Proteasomal degradation assays Samples containing 1 μg p15, in the absence or presence of PCNA at 1:5 molar ratio (12.5 μg) or BSA at 2.2 molar ratio (12.4 μg, Sigma-Aldrich) were incubated with 2 μg human 20S proteasome subcomplex (Enzo Life Sciences) at 37 °C in 16 μl of 30 mM Tris-HCl, pH 7.6, 100 mM NaCl, 10 mM CaCl 2 , 2 mM MgCl 2 , 1 mM DTT, 5% (v/v) glycerol. The reaction was stopped after 1, 2 or 4 h by adding gel loading buffer and boiling. Samples were run on a precast SDS–PAGE gel (4–12% gradient, Invitrogen) and stained with Coomassie Brilliant Blue. The remaining p15 was quantified by densitometry. Assuming that p15 can only be degraded after dissociating from PCNA, the degradation mechanism can be described by a simple two-step reaction (dissociation from PCNA, then degradation): The maximal degradation rate is given by the measured first-order rate constant for free p15 ( k deg =5.5 × 10 −4 s −1 , Fig. 4b ). Degradation of p15 may be assumed to be the rate-limiting step, considering that the dissociation constant is in the low micromolar range and that the binding to PCNA does not induce major structural rearrangements in either partner. For comparison, the dissociation rate constant of the p21–PCNA complex measured by surface plasmon resonance is k off =6.2 × 10 −4 s −1 at 37 °C (ref. 57 ). Taking into account that the affinity of p21 for PCNA exceeds that of p15 by three orders of magnitude and that the stoichiometry of binding to PCNA is 1:1 for both, it can be expected that k off of p15 largely exceeds its intrinsic k deg . With this assumption, the concentration of p15 that remains non-degraded by the proteasome at time t can be calculated from the following equation: where [p15] 0 is the initial concentration of p15 and [p15] free is the concentration of free p15, which can be calculated using the dissociation constant at 37 °C ( K d =3.3 μM). The equation was numerically solved assuming that [p15] free is invariant within infinitesimally small intervals and the reaction follows a zero order kinetics, where [p15] decreases linearly with time. The remaining p15 at each reaction time was derived by iteratively recalculating [p15] 0 and [p15] free in steps of 1 s (smaller time intervals yielded the same protein concentrations within <0.1% deviation). Figure 4b shows the calculated degradation curve together with the maximal uncertainty derived from the estimated errors in protein concentration (10%) and dissociation constant (10%), and the fitting error in the degradation rate of free p15 (0.06 × 10 −4 s −1 ). Electron microscopy PCNA at 0.1–0.025 g l −1 was mixed with a 1:6 molar excess of p15, 1:12 molar excess of dsDNA, or both (in PBS, pH 7.0, 1 mM DTT). The samples were applied to glow-discharged carbon-coated copper grids and stained with 1% (w/v) uranyl formate. Micrographs were taken at low radiation dose on a Jeol JEM-1230 LaB 6 transmission electron microscope operated at 100 kV and equipped with an Orius SC1000 CCD camera. More than 100 micrographs with a nominal magnification of 30,000 (2.3 Å per pixel) were recorded per sample. Sets of 8,759, 4,277 and 5,343 particles of the p15–PCNA–DNA, p15–PCNA and PCNA–DNA samples, respectively, were manually selected and windowed using XMIPP [58] . These sets were subjected to an iterative process of reference-free two-dimensional alignment and classification using the CL2D algorithm of XMIPP. An independent analysis was done for each of the three data sets based on the rotational power spectra of each individual particle, which were classified using a 7 × 7 or 10 × 10 Kernel probability Density Estimator Self-Organizing Map (KerDenSOM) classificatory matrix [59] . Coordinates and structure factors of the p15–PCNA complex are deposited in the Protein Data Bank under accession code 4D2G . The assignment of p15 bound to PCNA is deposited in the BioMagResBank with accession code 19868. How to cite this article: De Biasio, A. et al. Structure of p15 PAF –PCNA complex and implications for clamp sliding during DNA replication and repair. Nat. Commun. 6:6439 doi: 10.1038/ncomms7439 (2015).